Relativistic electron avalanches as a thunderstorm discharge competing with lightning Gamma-ray ‘glows’ are long duration (seconds to tens of minutes) X-ray and gamma-ray emission coming from thunderclouds. Measurements suggest the presence of relativistic runaway electron avalanches (RREA), the same process underlying terrestrial gamma-ray flashes. Here we demonstrate that glows are relatively a common phenomena near the tops of thunderstorms, when compared with events such as terrestrial gamma-ray flashes. Examining the strongest glow measured by the airborne detector for energetic emissions, we show that this glow is measured near the end of a downward RREA, consistent with occurring between the upper positive charge layer and the negative screening layer above it. The glow discharges the upper positive layer by ≥9.6 mA, strong enough to be an important charging mechanism of the storm. For this glow, the gamma-ray flux observed is close to the value at which relativistic feedback processes become important, with an avalanche multiplication factor of 4,500. The relativistic runaway electron avalanche (RREA) process was first proposed by Gurevich et al. [1] to help explain the large flux of gamma rays seen by McCarthy and Parks [2] in 1983 aboard a NASA F-106 airplane during a thunderstorm. Since then, several groups have measured glows from the ground [3] , [4] , [5] , [6] , [7] and from balloons [8] , [9] . Other groups refer to glows as thunderstorm ground enhancements (TGE) (ref. 10 ) and gamma-ray background growth (GRB) (ref. 11 ). The glow phenomenon follows from Wilson’s hypothesis [12] that energetic electrons in an electric field, such as those in thunderclouds, could accelerate to relativistic velocities even in fields where thermal electrons cannot overcome atmospheric friction. These seed electrons, slightly to significantly relativistic, are created as cosmic ray secondaries. For the RREA mechanism, Gurevich et al. [1] considered the effect of Møller scattering. In this scenario, relativistic electrons elastically scatter with other electrons, thereby producing an avalanche of relativistic electrons. The electrons emit bremsstrahlung gamma rays as they slow down from interactions with air molecules. RREA is the generally accepted mechanism for explaining the incredibly bright and energetic terrestrial gamma-ray flashes (TGFs) that have been seen by satellites. The spectrum of gamma-ray glows is similar to that of TGFs [13] , [14] , [15] but is orders of magnitude less bright. To explain the brightness of TGFs, Dwyer [14] , [16] , [17] proposed the relativistic feedback mechanism. The relativistic feedback process builds on the RREA process by including the physics of backscattered gamma rays and positrons from gamma-ray pair production, both of which propagate to the start of the avalanche region and generate new avalanches, producing an exponential growth in the number of avalanches. As thunderclouds charge, RREA and therefore glows may produce a significant discharge current, which can balance the charging of the cloud, with the bulk of the current coming from molecules ionized by the relativistic particle, not the energetic electrons directly [18] . Lightning is one of the main mechanisms that can discharge thunderclouds [19] . While estimations of the conductivity induced by RREAs vary [20] , [21] , RREAs are thought to enhance the conductivity at least somewhat and might therefore help discharge the cloud [1] . We show that during gamma-rays glows, the electric field is approaching the levels necessary for feedback but the field is not high enough to produce a TGF. We demonstrate for the first time that glows can provide a comparably effective channel to lightning for thunderstorm discharge. Glows overview and modelling The airborne detector for energetic lightning emissions (ADELE) measured 12 gamma-ray glows during 9 flights and 37 flight hours in the Colorado and Florida region. ADELE flew on a National Center for Atmospheric Research (NCAR) Gulfstream V during August and September 2009. The maximum cruising velocity of the plane is 262 m s −1 . The glows were detected using two large 12.7 cm diameter, 12.7-cm-long plastic scintillators. Each detector was in a separate aluminium box with the top detector having lead lining the bottom half of the plastic scintillator and with the opposite configuration for the bottom detector. These detectors were read out by discriminators with energy thresholds corresponding to roughly 50 and 300 keV, and 1 and 5 MeV. These energies were verified using sealed gamma-ray source calibrations. We used a two stage Monte Carlo simulation to compare our results with the spectrum caused by RREA. The first stage propagates electrons generated by relativistic runaway through an exponential atmosphere at various altitudes. The Monte Carlo simulation includes all the relevant physics for describing energetic electrons and positrons along with the emission and propagation of energetic photons [18] , [22] . The second stage takes the gamma rays, electrons and positrons that pass through the Gulfstream V’s cruising altitude of 14.25 km and feeds their energy, trajectory and particle type through a GEANT3 (ref. 23 ) model of the plane and ADELE to simulate the observed count rate in each discriminator channel. As long as ADELE was directly within, above or below an avalanche, and not to the side, comparing the ratios of different discriminator channels and detectors in the data and model directly constrains ADELE’s position in the avalanche and the avalanche direction. ADELE observed 12 gamma-ray glows, 3 of which were double-peaked. A glow seen on 21 August is 20 times brighter than any other glow and therefore contains the best spectral information. Durations ranged from 4 to 112 s but these values, except for the 21 August glow, are most likely due to the plane’s motion rather than intrinsic variation, the spread being due to different sizes of the glow region and the varying lateral distance of the aircraft in each case. The 21 August glow ends abruptly and much too quickly to be due to anything other than a rapid, lightning-like discharge of the cloud although no lightning was simultaneously detected. This abrupt ending is similar to the glows measured by McCarthy and Parks [2] and Tsuchiya et al. [24] . The abrupt ending in the other groups’ glows were caused by lightning, verified by measurements, allowing us to believe that something similar terminated the 21 August glow. 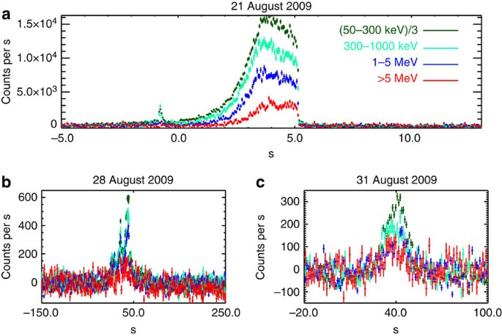Figure 1: Time profile of three ADELE glows. The two large plastic detector data have been summed and background subtracted. The lowest channel (dark green) is divided by three to show the higher energy channels more clearly. (a) The brightest glow on 21 August 2009, which had an abrupt ending; (b,c) two other more typical glows in which the instrument probably passed by but not through the avalanches. Figure 1 shows the 21 August glow compared with two other glows on different days, including all four energy channels. The significant counts in the >5 MeV channel rule out the spectrum of cold runaway emission from lightning leaders typically seen from the ground [25] . Figure 1: Time profile of three ADELE glows. The two large plastic detector data have been summed and background subtracted. The lowest channel (dark green) is divided by three to show the higher energy channels more clearly. ( a ) The brightest glow on 21 August 2009, which had an abrupt ending; ( b , c ) two other more typical glows in which the instrument probably passed by but not through the avalanches. Full size image Best-fit model for 21 august glow Taking the ratio of counts in the top and bottom detectors is not only useful for determining directionality, but is also sensitive to the fact whether bremsstrahlung gamma rays or the primary electrons themselves dominate the radiation field. The top/bottom ratio for 21 August increases over the four channels. The ratios for the four channels at the peak of the glow are 1.76±0.02, 1.71±0.04, 1.98±0.06 and 5.8+0.6/−0.5. These ratios are for the differential energy channels 50–300 keV, 300–1,000 keV, 1–5 MeV and >5 MeV. These high ratios can only be obtained in the simulations if ADELE is both directly in a downward avalanche and in the end of the avalanche, where the vast majority of particles are electrons rather than gammas. The increase of top/bottom ratio for the highest two channels is indicative of the large population of electrons being directed downward at the plane. The higher the energy of the electron, the more likely it will make it through the airplane exterior and interact with our detector. 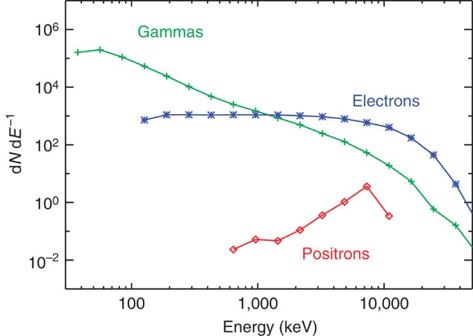Figure 2: Particle energy spectra for each particle type for the best-fit RREA model. This is the particle spectra at 14.25 km, the modelled flight altitude of the Gulfstream V. The end of the avalanche, which is directed downward, is at 14 km. Figure 2 shows the energy spectrum for each particle type for the best-fit RREA model at the elevation of the Gulfstream V before it was run through the instrument and airplane model. Refer to Fig. 6 in the Methods section to see the energy spectrum after the airplane and instrument have been included. At higher energies, electrons begin to dominate the total spectrum and this plays a very significant role in hardening the observed spectrum and creating large top/bottom ratios in ADELE’s higher energy channels. Figure 2: Particle energy spectra for each particle type for the best-fit RREA model. This is the particle spectra at 14.25 km, the modelled flight altitude of the Gulfstream V. The end of the avalanche, which is directed downward, is at 14 km. Full size image Figure 6: The difference between the ADELE data and various versions of the model. Different source altitudes and charge structures are shown in each plot. In all plots, the black dots are the data. 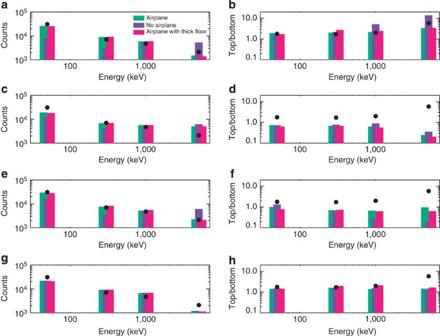Figure 6: The difference between the ADELE data and various versions of the model. Different source altitudes and charge structures are shown in each plot. In all plots, the black dots are the data. Plots on the left show the spectrum while plots on the right show the top/bottom ratio as a function of energy channel. Error bars for the data points are smaller than the plotting symbol. (a) The spectrum of 14 down models and data. (b) Top/bottom for 14 down and data. (c) The spectrum of 12 down models and data. (d) Top/bottom for 12 down and data. (e) The spectrum of 16 up models and data. (f) Top/bottom for 16 up and data. (g) The spectrum of 16 down and data. (h) Top/bottom for 16 down and data. Plots on the left show the spectrum while plots on the right show the top/bottom ratio as a function of energy channel. Error bars for the data points are smaller than the plotting symbol. ( a ) The spectrum of 14 down models and data. ( b ) Top/bottom for 14 down and data. ( c ) The spectrum of 12 down models and data. ( d ) Top/bottom for 12 down and data. ( e ) The spectrum of 16 up models and data. ( f ) Top/bottom for 16 up and data. ( g ) The spectrum of 16 down and data. ( h ) Top/bottom for 16 down and data. 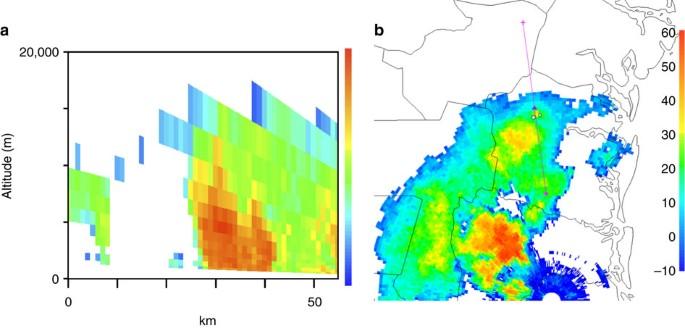Full size image The simulations show that the hardness of the spectrum for the 21 August glow is consistent with being within the avalanche region, and not just the gamma-ray field above it. Figure 3: Reflectivity during the ADELE glow. (a) The vertical cross-section of reflectivity (in dBZ) along the line shown in the right panel. (b) The horizontal cross-section of reflectivity (in dBZ). The two small white boxes mark the position of the Gulfstream V at the beginning and end of the glow. Figure 3 shows a radar reflectivity created using the Unidata IDV software [26] . Weather Surveillance Radar—1988 Doppler (WSR-88D) level II (base) data for Jacksonville, Florida was obtained from the National Climatic Data Center (NCDC). For the altitude of 14.1 km that the Gulfstream V was flying during the 21 August glow in conjunction with the top/bottom ratio and spectral information, and if we assume a simple cartoon tripolar model of a thundercloud [19] , it is consistent that ADELE was flying between the upper positive charge centre and its negative screening layer. The radar data indicate that the altitude of 14.1 km is close to the top of the cloud, a little below where one would expect the negative screening layer to be [19] , [27] . Being in this region of the cloud allowed ADELE to measure a glow from within the avalanche. It seems likely that the factor of 20 intensity difference between this glow and the others is that the other glows were observed only in the gamma-ray radiation field, above and laterally displaced from the avalanche itself; this is supported by the flight path data and lightning maps for the other glows. Figure 3: Reflectivity during the ADELE glow. ( a ) The vertical cross-section of reflectivity (in dBZ) along the line shown in the right panel. ( b ) The horizontal cross-section of reflectivity (in dBZ). The two small white boxes mark the position of the Gulfstream V at the beginning and end of the glow. Full size image Approaching relativistic feedback during peak ice From the peak brightness observed, we can conclude that the cloud was approaching the limit necessary for feedback for the electric field modelled, 400 kV m −1 at sea level, typical for a thunderstorm [18] . This is equivalent to an electric field of 67.6 kV m −1 at 14.1 km. Gurevich et al. [1] suggested that the maximum field or breakeven field is between 200 and 400 kV m −1 at sea level. Fields can commonly surpass the breakeven field but these high fields are usually accompanied by lightning [28] . The Monte Carlo simulation of our instrument gives the counts in a detector per electron per unit area that were used in the simulation. Normalizing the results of our GEANT simulation by dividing the observed counts by the simulated counts per electron per unit area, we can find the electron flux at the observed altitude. To find the flux at the end of the avalanche, we use the altitude variation in the model to extrapolate; in this case, the extrapolation is small since we were near the end of the avalanche already. We find the runaway electron flux at the end of the avalanche to be 1,100 electrons per s per cm 2 . From Carlson et al. [29] , we assume a 1 MeV seed electron flux of 0.25 counts per s per cm 2 from the cosmic ray background. This is an avalanche multiplication factor of 4,500, close to but still <5,000, where feedback begins to dominate [22] . Our systematic uncertainty due to limited information about the aircraft mass distribution allows the range of electron flux to be 750–1,400 electrons per s per cm 2 and the range of avalanche multiplication factors to be 3,000–5,600. The density and size of ice particles were measured by the NCAR cloud droplet probe (CDP) during the ADELE flights. 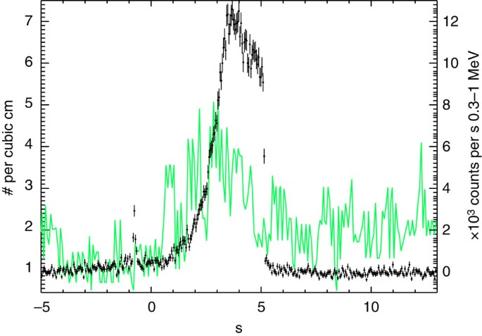We believe the cloud particles to be all ice since the ambient temperature was −68 °C during the glow. Figure 4: Ice concentration during glow. The small ice particle concentration in the range of 2–60 μm diameter (green) as measured by the CDP against the count rate for the 21 August glow (black) as a function of time. Figure 4 shows the small cloud particle (between 2 and 60 μm) concentration alongside the 21 August glow. The average and median particle size detected by the CDP during the glow is about 40 μm. During the glow there was a large spike in the small ice concentration. The NCAR two-dimensional cloud probe, which is sensitive to particles between 50 and 1,000 μm, shut down during the glow after it began to measure very high concentrations of large ice. Figure 4: Ice concentration during glow. The small ice particle concentration in the range of 2–60 μm diameter (green) as measured by the CDP against the count rate for the 21 August glow (black) as a function of time. Full size image Because gamma-ray glows persist for seconds to minutes [30] , [31] , most of the discharge current resulting from runaway electrons will come from the drifting ions and not the low-energy electrons or runaway electrons [16] . In the runaway electron avalanche region, the main source of ions is the ionization caused by the runaway electrons. Each runaway electron creates α electron–ion pairs per unit length by ionizing the air. The low-energy electrons then attach to oxygen on the timescale of microseconds, forming negative ions. If we assume that the density of ions is not too large, ion–ion and ion–electron recombination may be ignored. The main loss of ions is then assumed to be attachment of ions to cloud ice and water particles. The temperature of air during the glow was −68 °C so we can assume that all water was in the form of ice. The attachment length, λ cl , depends on the density of cloud particles, the total water content, the charge on the cloud particles and the electric field [19] , [32] , [33] . The CDP is not designed to measure non-spherical ice, but if we assume a particle density of roughly 10 particles per cm 3 and a particle diameter of 40 μm, which is consistent with both the CDP measurement during the glow and the literature for similar meteorological situations [34] , [35] , [36] , we find λ cl to be 27 m. The value of 10 particles per cm 3 was chosen to be conservative by a factor of 2 compared with the numbers shown in Fig. 4 when calculating the discharge current. For simplicity, we shall assume that this length is the same for positive and negative ions. The density of positive and negative ions, n ± , is then given by where F re is the flux (particles per m 2 per s) of runaway electrons; the ionization per unit length, α ∼ 8,350/m × N , where N is 0.169, the density of air relative to that at standard conditions [21] ; μ ± is the mobility of the ions where μ + =(1.4 × 10 −4 m 2 V −1 s)/N and μ − =(1.9 × 10 −4 m 2 V −1 s)/N [37] ; and E is the electric field strength. In the steady state, which should apply to glows, Using equation (2), the electric current produced by the drifting positive and negative ions is For the observed runaway electron flux of 1.1 × 10 7 electrons per s per m 2 , this gives a discharge current density of ∼ 130 nA m −2 . For the range of electron flux due to uncertainty of the airplane mass distribution, the range of possible current densities is 90–170 nA m −2 . These are comparable to other thunderstorm discharging currents, such as lightning and precipitation [19] . Positive intracloud (+IC) and positive cloud-to-ground (+CG) lightning are the types responsible for discharging the upper positive charge region of a thunderstorm. Using the US Precision Lightning Network (USPLN) and estimations to get the true IC flash rate based on the CG flash rate [38] , [39] , we look at +CG and IC lightning in the same cell as the glow during a ±10-min duration of the glow. We find that lightning discharged the upper positive region of the cloud between 33 mA and 1.0 A, while the glow discharged the same region with a mean current in the range 9.6 mA and 3.3 A. The range covers area estimates for the glow with varying assumptions, giving 1 km 2 , 6.4 km 2 and 26 km 2 (see Methods), and glow duty cycle from 8 to 100% (see below). The frequency of glows that ADELE observed at cruise altitude—despite not passing directly through as on 21 August—demonstrates that the glow discharge process is not rare or anomalous, especially when compared with TGFs [40] . All of the other glows, except one, occurred when the Gulfstream V was passing near an active lightning cell. Glows were observed 11 out of the 149 times that ADELE was close to an active electrified storm. This allows us to place a lower limit on the frequency of glows, that roughly 8% of electrified storms produce glows, but that value is extremely conservative. Glows may in fact be much more common because glows turn on and off with electrification of the storm [2] , [30] so ADELE may not have been passing by a cell when the glow was ‘on’. ADELE also may not have been close enough to the electrified storms to successfully measure a glow. The altitude difference—and, even more strongly, any lateral distance—between the storm and the instrument will cause attenuation of gamma rays and make many of the glows produced in these cells, if they exist, too faint to measure. The policy during this campaign was to not fly directly into thunderstorms, as a safety precaution. However, this was accidentally breached once during the 2009 campaign. This is when the bright glow on August 21 was measured. The brightest gamma-ray glow observed implies that RREA current played a significant role in that cloud’s discharging. We find that glows may play an important role in the overall charge balance of thunderstorms, and perhaps electrified shower clouds, which by definition do not use lightning to discharge. All observed glows agree with the RREA spectrum; the glow on 21 August, however, showed that sustained RREA can happen at a flux level requiring feedback. The glow spectrum from each of our large plastic detectors on 21 August was consistent with a large population of energetic electrons above the plane and the gamma rays from bremsstrahlung below the plane. This geometry implies that ADELE is in the end of the avalanche region with the avalanche downward facing, and therefore possibly flying between the main upper positive and negative screening layer. ADELE is an array of gamma-ray detectors that was originally designed to study TGFs from a plane. During its first campaign, it measured 12 gamma-ray glows and 1 TGF. We discuss the methods used for acquiring, processing and analysing our glow data. The brightest glow on 21 August was analysed most extensively and the uncertainties in modelling are addressed here. The 2009 ADELE flight campaign In 2009, ADELE consisted of two sensor heads, each with three scintillators, a plastic and NaI cylinder each 12.7 cm in diameter and 12.7-cm-long and a plastic cylinder with a 2.54 cm diameter and 2.54 cm length, all read out by photomultiplier tubes. In the top sensor head, a 0.32 cm lead shield was placed along the bottom of each scintillator allowing those detectors to be more sensitive to radiation coming from above. The opposite was done in the bottom sensor head, allowing the ratio of the top/bottom counts to give directionality. Signals from the plastic scintillators’ photomultiplier tubes are sent to fast-chain electronic boards containing discriminators at four energy thresholds, ∼ 50 and 300 keV, and 1 and 5 MeV. The discriminator outputs are sent to a field-programmable gate array (FPGA) where counts (rising edges) and deadtime fraction are accumulated in 50 μs bins for every channel. The output from the NaI detectors was recorded only in a triggered mode that was not used in this work. The instrument configuration is shown in Fig. 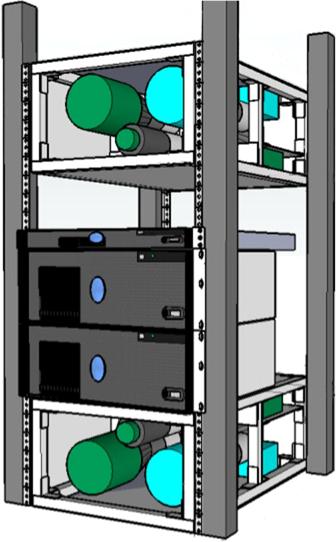5 . Figure 5: The ADELE schematic. The green detectors are plastic while the turquoise detector is NaI. The two black rectangular boxes are the two computers, while the thin black box above the computers is the electronics tray. These are all mounted into a rack as shown. Figure 5: The ADELE schematic. The green detectors are plastic while the turquoise detector is NaI. The two black rectangular boxes are the two computers, while the thin black box above the computers is the electronics tray. These are all mounted into a rack as shown. Full size image ADELE flew aboard a Gulfstream V operated by NCAR during August and September 2009. The flights took place over regions near Colorado and Florida. During the 37 h of flight that ADELE was onboard, 12 gamma-ray glows were seen, with some glows reappearing during multiple passes of the plane over the same cell. After binning the counts of the large plastic detectors into 2-s bins, the data were visually searched for glows. Glows were defined as series where the counts increased for >2 s. To ensure that we were not observing count rate changes due to altitude fluctuations of the airplane, a relationship between altitude and count rate was found during the ascent of the plane between 10 km and the cruising altitude (between 14 and 15 km). The effects from altitude were removed from all count rates. ADELE modelling and uncertainties To model the glow on 21 August, which was over 20 times brighter than any other glow in our data, we used a model of relativistic runaway avalanches with positron and gamma-ray feedback [18] , [22] . The electric field was not measured directly but was modelled to be 400 kV m −2 (equivalent at sea level) with a vertical extent of 68.72 g cm −2 and a large horizontal extent. The output from this stage includes gamma rays, electrons and positrons along with their energies and trajectories. These are then fed into a GEANT3 model [23] that replicates the detectors, sensor heads, computers and electronics of the ADELE instrument and places them in a large aluminium cylinder that represents the Gulfstream V fuselage. Unfortunately, the exact mass distribution of the Gulfstream V is not known. This affects the top/bottom ratios and, less significantly, the energy spectra that are given by our models. To account for this, we have modelled several extreme test cases to make sure our results are robust with the uncertainty. These include modelling an aluminium fuselage that is 40% of the total mass of the empty plane, no fuselage at all and extra aluminium mass below the instrument. These simulations along with our understanding of the Gulfstream V were used to determine the range of values for the avalanche electron flux, 750–1,400 electrons cm −2 s −1 . Figure 6 shows these three situations for four different RREA geometries: downward facing RREA with the end of the avalanche at 14 km, downward RREA at 12 km, upward RREA at 16 km and downward RREA at 16 km. For each of these RREA geometries, the spectral models and top/bottom ratios are compared with the data. The first three RREA geometries are physically plausible (within realistic thunderstorm charge structure) and show spectral models that roughly agree with the actual spectrum. However, 12 km down and 16 km up can be ruled out as viable options when the top/bottom ratio is taken into account. Sixteen kilometre down was included in this plot because it is a model that is dominated by gamma rays, since by the time it reaches the airplane the electrons have been lost. Comparing 16 km down to the three other models shows the effect that the electrons have on hardening the energy spectrum. The detector response is shown in Fig. 7 . The curves are for mono-energetic particles coming directly from above the aircraft. We do not use these responses directly, since we inject a complete avalanche model directly into our instrument in our simulations. For input angles even slightly off the vertical, the lower detector will have a bigger response because the lower detector is no longer completely shadowed by the top detector and the lead shield beneath it. 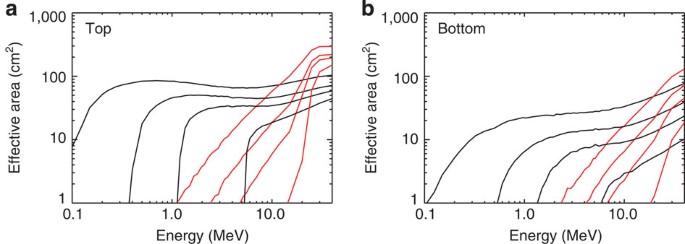Figure 7: The ADELE detector response for the large plastic scintillators. The effective area as a function of photon or electron energy is shown for monoenergetic particles coming from above the top detector (a) and bottom detector (b). Red curves represent electrons and black curves gamma rays. Each set of four curves represents the rate in one of the integral energy channels, from left to right >50 and >300 keV, and >1 and >5 MeV. Figure 7: The ADELE detector response for the large plastic scintillators. The effective area as a function of photon or electron energy is shown for monoenergetic particles coming from above the top detector ( a ) and bottom detector ( b ). Red curves represent electrons and black curves gamma rays. Each set of four curves represents the rate in one of the integral energy channels, from left to right >50 and >300 keV, and >1 and >5 MeV. Full size image Comparing glow current with nearby lightning current To compare the amount of current moved by the glow to the total current moved by the lightning during the same period, the size of the cell needs to be approximated. Using an echo at an altitude of >12 km, the size of the overshooting top, depending on a threshold reflectivity, was estimated to be between 6.4 and 25.7 km 2 . However, the true lower limit on the size of the glow is about 1 km 2 . This comes from the speed of the Gulfstream V and the amount of time ADELE spent passing through the peak of ice. To calculate the amount of current that lightning moved during the brightest glow on 21 August, lightning within the largest cell of the glow (26 km 2 ) and within 20 min of the glow was used. The lightning was detected by the USPLN. About 15 −CG flashes and 1 +IC flash were detected in the largest box, and since the lightning was occurring uniformly throughout the region we use these numbers to scale the current down based on the ratios of areas in the smaller boxes to give us better statistics. If we assume that the glow occurred between the upper positive and negative screening layer, the only types of lightning that could deplete that charge region are +IC and +CG flashes. We take typical values for the charge carried by +IC flashes [41] of 20 C and by +CG flashes [42] of 80 C. USPLN is much more sensitive to CG flashes than IC flashes, so two methods were used to estimate the true number of IC flashes. From Pierce [38] , we can use to determine the ratio of IC to CG flashes, where λ is latitude in radians. The currents from the largest box (26 km 2 ) were scaled down to the smaller boxes (1 and 6.4 km 2 ). This yields currents of 33, 210 and 840 mA for the three area guesses of the cell. The other method was from Prentice and Mackerras [39] , the ratio of IC to CG is given by , also with λ as latitude in radians. The discharge current from that ratio is 40 mA, 260 mA and 1.0 A. So the total current within 20 min of the glow in the same cell as the glow was between 33 mA and 1.0 A depending on the size of the cell and the method used for determining IC flashes. To find the amount of current moved by the glow, we assume a glow discharge rate of 130 nA m −2 and the same areas assumed above. There is an uncertainty in the glow discharge rate of about 30% due to uncertainties of the mass distribution of the plane (see above subsection). While we measured the glow for only 4 s, it is reasonable to assume the glow was active for much longer since groups on the ground measure glows for several minutes [31] , [43] . From the rest of our glow measurements, we know that glows are occurring near active storm cells at least 8% of the time. Glows are probably much more common but were not measured because of our flight rules of not passing into active thunderstorm regions. Using the same ±10 min of the time when ADELE measured the glow as was used in the lightning comparison, we can find the upper and lower limit for the amount of current produced by this glow. The lower limit assumes that it is only glowing for 8% of the 20 mins and uses the smallest cell size while the upper limit assumes it was glowing the entire time and uses the largest cell size. This creates the range of 9.6–130 mA for the 1 km 2 cell size, 60–810 mA for the 6.4 km 2 cell size and 270 mA–3.3 A for the 26 km 2 cell size. The true amount of current moved would be somewhere between those amounts. While these calculations are just approximations, the qualitative conclusion is that glows produce a significant amount of discharge current (comparable to lightning) and should be considered when taking into account the overall charging and discharging dynamics of a thundercloud. How to cite this article: Kelley, N. A. et al. Relativistic electron avalanches as a thunderstorm discharge competing with lightning. Nat. Commun. 6:7845 doi: 10.1038/ncomms8845 (2015).